Loss-proof self-accelerating beams and their use in non-paraxial manipulation of particles’ trajectories Self-accelerating beams—shape-preserving bending beams—are attracting great interest, offering applications in many areas such as particle micromanipulation, microscopy, induction of plasma channels, surface plasmons, laser machining, nonlinear frequency conversion and electron beams. Most of these applications involve light-matter interactions, hence their propagation range is limited by absorption. We propose loss-proof accelerating beams that overcome linear and nonlinear losses. These beams, as analytic solutions of Maxwell’s equations with losses, propagate in absorbing media while maintaining their peak intensity. While the power such beams carry decays during propagation, the peak intensity and the structure of their main lobe region are maintained over large distances. We use these beams for manipulation of particles in fluids, steering the particles to steeper angles than ever demonstrated. Such beams offer many additional applications, such as loss-proof self-bending plasmons. In transparent media these beams show exponential intensity growth, which facilitates other novel applications in micromanipulation and ignition of nonlinear processes. Since the first demonstration of self-accelerating optical beams in 2007 by Siviloglou and Christodoulides [1] , [2] , the field has attracted considerable attention from both theoretical and applicative points of view. Chronologically, the first of such beams was the Airy beam, relying on an earlier discovery by Berry and Balazs who have found a self-accelerating solution to the Schrödinger equation [3] . This Airy solution, which is propagating on a parabolic trajectory, relies on the mathematical equivalence between the Schrödinger equation and the paraxial wave equation for electromagnetic waves. The tendency of the Airy beam to maintain an invariant intensity profile while bending its propagation direction enabled interesting applications such as optical micromanipulation of particles [4] , [5] , microscopy [6] , [7] , laser machining of curved structures [8] , generation of curved plasma channels in the air [9] , self-bending electron beams [10] and control of plasmonic surface waves [11] , [12] , [13] . The field has taken a substantial step forward when accelerating solutions of the full Maxwell equations were introduced [14] . These beams support bending of light beams to large angles, up to almost 180°, rather than the Airy beam that can only bend up to ~10° before breaking the paraxial approximation. Such non-paraxial accelerating beams were demonstrated experimentally soon thereafter [15] , [16] , [17] . Likewise, several other types of accelerating beams, such as Weber and Mathieu beams, were discovered [18] , [19] , [20] , as well as nonlinear paraxial [21] , [22] , [23] , [24] and nonparaxial [16] , [25] accelerating beams, and even accelerating beams in curved space [26] . All of these beams exhibit similar features—diffractionless propagation, transverse acceleration and self-healing, which allows the beam to rebuild itself after going through partial blocking or distortion. It is now clear that the major interest generated by accelerating electromagnetic beams is caused by their ability to interact with matter: exert forces on particles, induce plasma channels in air, trigger self-bending plasmonic wavepackets, and so on. Many of these naturally involve loss due to absorption [9] , [12] , [13] , which limits the propagation range of the bending beams. For example, the creation of Airy plasmons has shown very limited propagation distances and distortion of the beam shape due to heavy losses in the metal–dielectric interface. Likewise, in optofluidic and biological applications, the optical beams often propagate in absorbing liquids, which attenuate the beam and make the optical functionality difficult or impossible. Of course, the problem of absorption is not restricted to accelerating beams—it is a limiting factor for all optical beams and applications. For example, the propagation range of optical solitons—nonlinear waves that propagate while maintaining their shape by balancing diffraction with nonlinear focusing effects—is also limited by loss, because as power is absorbed, the nonlinearity decreases and can no longer balance diffraction. Generally speaking, the issue of absorption in optics is usually only dealt with via external means (for example, amplifiers or appropriate sample design), and presently there are no generic optical beams that can maintain the peak intensity value and the structure of their main lobe in lossy media. Several avenues to overcome this limitation have been demonstrated [27] , [28] , [29] , [30] , but none targeted shape-preserving accelerating beams. In this article, we introduce analytic loss-proof accelerating solutions of the full Maxwell equations in two dimensions: optical beams that can propagate through absorbing media while maintaining the intensity (value and structure) of their main lobe, for an arbitrarily long distance. This is achieved through the property of self-healing of nondiffracting beams, which allows energy transfer from the oscillating tail of the beam to the main lobe region. We exploit this property to predesign the beam so as to compensate for the loss, thereby making up for linear or nonlinear losses caused by the medium. Moreover, the loss-proof concept presented here for beams evolving on circular trajectories [14] can be readily introduced for shape-preserving accelerating beams of other kinds of trajectories, for example, beams propagating on elliptic or parabolic trajectories [18] , [19] , [20] , and even for beams that follow arbitrary trajectories [32] , [32] . As such, the ideas can be used for loss-proof propagation for arbitrarily large distances. Such beams can be used to create loss-proof long-range plasmons and manipulate particles in absorbing fluids, especially in biological fluids. Naturally, the paraxial limit of our solutions yields loss-proof Airy beams, which were not known before, and should have a variety of applications as well. Moreover, when propagating in vacuum or in lossless media, the loss-proof beams display exponential growth in peak intensity, which can be used for acceleration of particles, ignition of intensity-driven nonlinear processes or serve as a controllable focus light source. We present these beams here theoretically and experimentally, and demonstrate their use in micromanipulation of particles within a fluid. Importantly, these experiments utilize non-paraxial accelerating beams, demonstrating circular acceleration of microparticles at much steeper angles than ever achieved by optical means. Loss-proof beams of Maxwell’s equations We begin by examining Maxwell’s equations in a linear, homogenous and isotropic material, with conductance σ : For convenience, we express all linear losses through the Ohmic conductance, which accurately describes the loss in plasmonic media. In dielectrics, where losses represent absorption by electric dipoles, the loss can be cast into an Ohmic term and appear in the same fashion in the Helmholtz equation. From here we derive the wave equation in lossy media We focus in this paper on two-dimensional solutions. Thus, we first seek TE-polarized solutions of the form . Equation (2) has full symmetry with respect to x and z , hence we expect a circular trajectory, similar to ref. 14 . Exploiting this symmetry, we seek shape-preserving solutions propagating on a circular trajectory. To do this we transform our equation into polar coordinates with z = r sin θ , x = r cos θ : We seek solutions with radial symmetry of the form , where α is some real number and ω is the wave frequency. U ( r ) must satisfy The exact solution for this equation is the Bessel function of order α and complex argument: where are the real and imaginary parts of the wavevector, respectively. These parameters are determined by setting the initial conditions on the beam and are chosen to match the real and imaginary parts of the refractive index, such that the beam ‘heals itself’ exactly at the correct rate. We are interested only in the forward-propagating beam, hence we take only the forward-propagating part of the Fourier spectrum, which yields the ‘half-Bessel’ solution known from ref. 14 , but with a complex argument: The main difference between this solution and the non-paraxial accelerating beam found in ref. 14 is in the diverging tail of the loss-proof beam found here. In a similar manner, one can find the loss-proof accelerating TM solution, as was done for the lossless case in ref. 14 . Having found both TE and TM solutions, this leads to full vectorial loss-proof accelerating solutions, similar to the vectorial solutions in the lossless case [19] , [33] . Keeping in mind that the accelerating beams, paraxial (Airy) and non-paraxial, are not square-integrable, the fact that this loss-proof accelerating beam has a diverging tail is intriguing but does not pose any physical problems more than the other accelerating beams do. Namely, as with all other accelerating beams, the Fourier spectrum would have to be truncated (with some apodization). Therefore, the range at which this beam remains shape-preserving would also be finite, but it is nonetheless much greater than the absorption length in the lossy medium. When propagating in a lossy medium, the increased power transfer from the tail to the front lobes makes up for the absorption and preserves the lobes at a constant intensity. The loss-proof effect can be viewed as an intensified self-healing process: tail lobes of higher intensity transfer more power to the front lobes, and maintain the intensity of the main lobe (value and structure) despite the loss. Comparison with ordinary accelerating beams A comparison between the loss-proof beam and an ordinary accelerating beam, both propagating in the same lossy medium, is depicted in Fig. 1 . 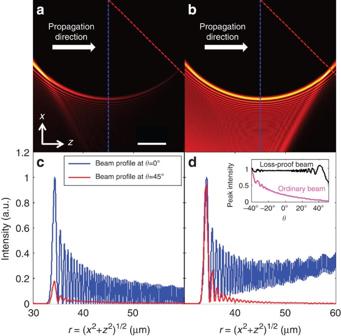Figure 1: Loss-proof non-paraxial accelerating beam compared with an ordinary accelerating beam. (a) Dynamics of an ordinary non-paraxial accelerating beam (α=400, wavelength 532 nm) propagating through an absorbing medium with absorption coefficientk″=k′/500. The beam maintains its shape but its intensity decays during propagation. Scale bar, 10 μm. (b) Dynamics of a loss-proof non-paraxial beam propagating through the same medium and launched from the same aperture. In this case, the intensity of the main lobe remains invariant during propagation, while the tail decays to compensate for the losses. All parameters are identical toa. (c,d) Profiles of the beams ofaandbtaken at the blue and red planes therein, which correspond to bending ofθ=0° andθ=45°. Inset: Comparison between the peak intensity of the main lobe of the ordinary accelerating beam ofaand that of the loss-proof accelerating beam ofb, as the beams propagate on the same trajectory. The beams start off with the same peak intensity, but the ordinary accelerating beam decays exponentially in intensity due to absorption, whereas the loss-proof beam maintains its peak intensity over more than 80° of bending. Figure 1a shows the propagation of an ordinary non-paraxial self-accelerating beam designed for lossless media, , with Fig. 1c displaying two cross-sections of the beam as it is propagating: at θ =0° and at θ =45°. As expected, this beam maintains its shape but its intensity decays exponentially during propagation. On the other hand, the loss-proof accelerating beam depicted in Fig. 1b maintains both the shape and the intensity of its main lobe during a 90° bending inside the absorbing medium. Figure 1d displays this by showing the cross-sections of the loss-proof beam at θ =0° and at θ =45°. Note that the "tail" of the beam has an essential oscillatory envelope in Fig. 1d . This is caused by the truncation of the backward-propagating wave, and is also present in the ordinary beam in Fig. 1c and in ref. 14 , although less noticeable. The inset in Fig. 1 shows the peak intensity of both accelerating beams—ordinary and loss-proof—during propagation, starting at the same peak intensity. Evidently, the ordinary beam decays exponentially in intensity, while the loss-proof beam maintains its peak intensity along more than 80° of bending, despite the loss in the medium. For some applications, one would also like to compare the loss-proof accelerating beam and the ordinary accelerating beam under the same input power and the same aperture. Such a comparison is shown in Supplementary Fig. 2 and discussed in the Supplementary Information section, with a specific example showing a loss-proof beam that displays an improvement of 50% in the acceleration range over the ordinary beam of the same power, emitted from the same aperture and accelerating on the same curved trajectory. Figure 1: Loss-proof non-paraxial accelerating beam compared with an ordinary accelerating beam. ( a ) Dynamics of an ordinary non-paraxial accelerating beam ( α =400, wavelength 532 nm) propagating through an absorbing medium with absorption coefficient k ″= k ′/500. The beam maintains its shape but its intensity decays during propagation. Scale bar, 10 μm. ( b ) Dynamics of a loss-proof non-paraxial beam propagating through the same medium and launched from the same aperture. In this case, the intensity of the main lobe remains invariant during propagation, while the tail decays to compensate for the losses. All parameters are identical to a . ( c , d ) Profiles of the beams of a and b taken at the blue and red planes therein, which correspond to bending of θ =0° and θ =45°. Inset: Comparison between the peak intensity of the main lobe of the ordinary accelerating beam of a and that of the loss-proof accelerating beam of b , as the beams propagate on the same trajectory. The beams start off with the same peak intensity, but the ordinary accelerating beam decays exponentially in intensity due to absorption, whereas the loss-proof beam maintains its peak intensity over more than 80° of bending. Full size image Exponentially growing and decaying beams Another interesting feature of the loss-proof beam described by equation (7) is its behaviour when propagating in lossless media ( σ =0), with a beam designed with k ″≠0. In this case, equation (6) for k ″ is no longer fulfilled, so that the beam is no longer a solution of equation (4). This results in an ‘over-healing’ effect, where the power transfer from the tail to the main lobe is excessive. The beam is still shape-preserving, but now the beam intensity is rising exponentially along the curve, at a rate defined by the value of k ″ for which the beam was designed: , where R = α / k ′ is the acceleration radius and θ =sin −1 ( z / R ) is the angle of bending. For many cases of interest, the initial aperture is chosen such that the shape-preserving acceleration occurs up to , in which case one can approximate . This ‘exponentially growing beam’ effect is shown in Fig. 2b,d , in comparison with an ordinary non-paraxial accelerating beam ( Fig. 2a,c ). This beam is now showing exponential growth in its intensity, which continues until the beam’s tail is all used up. Once the power in the tail has all been transferred to the main lobes, the beam decays quickly. The inset in Fig. 2 compares the peak intensity of the ordinary beam and the exponentially growing beam during propagation in a lossless medium (free space). Both beams carry the same total power. The growing beam starts with lower peak intensity, since most of the power is concentrated at the beam’s tail, but during propagation the main lobe grows and, as expected, reaches peak intensity higher than that of the ordinary accelerating beam. Some applications would require a main lobe that reaches the highest possible peak intensity at a certain pre-chosen distance, assuming a fixed beam power. In this case, the beam would be designed so as to overcompensate for the loss, as in Fig. 2 . Of course, this can only be effective up to some distance and should be optimized specifically for each scenario. 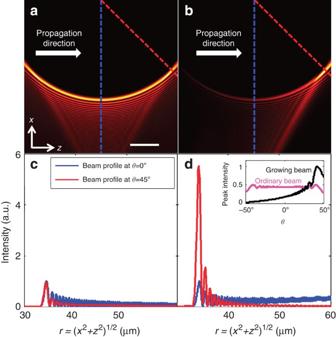Figure 2: Exponentially growing non-paraxial accelerating beam compared with an ordinary accelerating beam. (a) Dynamics of an ordinary non-paraxial accelerating beam in vacuum. The main lobe region of the beam maintains its shape and intensity throughout propagation. Wavelength and acceleration parameterαare the same as inFig. 1. Scale bar, 10 μm. (b) Dynamics of an exponentially growing non-paraxial accelerating beam in vacuum (launched from the same aperture asa). The intensity of the main lobe grows exponentially during propagation, as it is being overcompensated by power transfer from the tail. In this example, the intensity of the main lobe grows by almost factor 6. (c,d) Beam profiles atθ=0° andθ=45° for the ordinary and exponentially growing beams, respectively. Inset: Comparison between the peak intensity of the main lobe of the ordinary accelerating beam ofaand that of the growing accelerating beam ofb, as the beams propagate on the same trajectory. The beams start with equal total power, hence the growing beam starts with much lower peak intensity but then its peak intensity grows exponentially, reaching a higher peak intensity after a given propagation distance. Figure 2: Exponentially growing non-paraxial accelerating beam compared with an ordinary accelerating beam. ( a ) Dynamics of an ordinary non-paraxial accelerating beam in vacuum. The main lobe region of the beam maintains its shape and intensity throughout propagation. Wavelength and acceleration parameter α are the same as in Fig. 1 . Scale bar, 10 μm. ( b ) Dynamics of an exponentially growing non-paraxial accelerating beam in vacuum (launched from the same aperture as a ). The intensity of the main lobe grows exponentially during propagation, as it is being overcompensated by power transfer from the tail. In this example, the intensity of the main lobe grows by almost factor 6. ( c , d ) Beam profiles at θ =0° and θ =45° for the ordinary and exponentially growing beams, respectively. Inset: Comparison between the peak intensity of the main lobe of the ordinary accelerating beam of a and that of the growing accelerating beam of b , as the beams propagate on the same trajectory. The beams start with equal total power, hence the growing beam starts with much lower peak intensity but then its peak intensity grows exponentially, reaching a higher peak intensity after a given propagation distance. Full size image Loss-proof bending beams in media with nonlinear loss Importantly, our method for finding the loss-proof accelerating beams is not restricted to linear cases. For example, we also solve for loss-proof accelerating beams in media displaying nonlinear losses caused by two-photon absorption. This case is important for applications where multiphoton effects have a role, such as the curved plasma channel described in ref. 9 . A closely related example is using abruptly autofocusing beams (a cylindrical superposition of Airy beams) for multiphoton microscopy [34] , [35] . In such cases, where the losses stem from multiphoton absorption, proper design of the input beam can support an accelerating beam propagating for very large distances with its main lobe maintaining its structure and peak intensity in spite of the nonlinear losses. Let us illustrate this feature with an accelerating beam in a medium with two-photon absorption loss. The wavevector in this case can be approximated by , where | E | 2 is the beam intensity, β is the nonlinear absorption coefficient and . We substitute this into equation (4) to obtain In general, equation (8) can be solved for any nonlinearity, with either the real part of k (for example, Kerr or saturable), or the imaginary part of k (multiphoton absorption). We solve equation (8) and find the nonlinear self-accelerating loss-proof beams in a method similar to that of ref. 25 , which can be easily taken to the nonlinear paraxial limit discussed in ref. 21 . 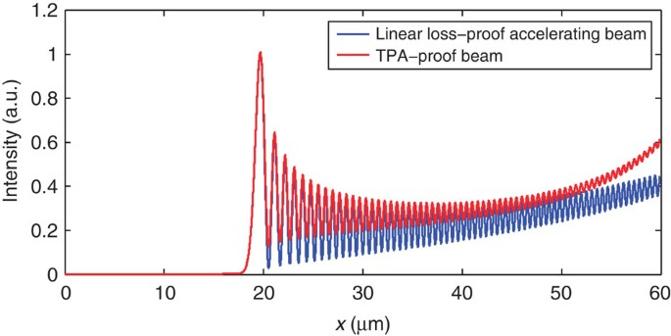Figure 3: Nonlinear loss-proof self-accelerating beam. The nonlinear beam (red) is designed to propagate without loss in a nonlinear medium where attenuation is caused by a two-photon absorption (TPA) process, with parametersμm W−1. For comparison, the linear loss-proof beam (blue) is designed to propagate in linearly absorbing medium, with parameters. Both beams have the same acceleration parameterα=120 and wavelengthλ=1 μm. Figure 3 compares the nonlinear and linear loss-proof solutions. The nonlinear beam (in red) is similar in shape to the linear case (in blue), but displays a different tail divergence rate, which is naturally defined by the losses. We emphasize that the method we use to find the loss-proof beams is very general, and other nonlinear cases, such as loss-proof beams in Kerr medium or the abruptly focusing beams mentioned earlier can be easily handled in a similar fashion. Figure 3: Nonlinear loss-proof self-accelerating beam. The nonlinear beam (red) is designed to propagate without loss in a nonlinear medium where attenuation is caused by a two-photon absorption (TPA) process, with parameters μm W −1 . For comparison, the linear loss-proof beam (blue) is designed to propagate in linearly absorbing medium, with parameters . Both beams have the same acceleration parameter α =120 and wavelength λ =1 μm. Full size image We demonstrate one application of loss-proof nondiffracting beams: extending the range of particle manipulation with accelerating beams. We create and image a loss-proof self-accelerating beam using a phase-only spatial light modulator (SLM) and an amplitude mask. In this setup, a continuous-wave laser source at wavelength 532 nm is used to illuminate a linearly polarized wide Gaussian beam upon the SLM, which imposes the appropriate Fourier space phase on the beam. While in previous experiments, phase-only modulation was sufficient to generate accelerating beams [2] , [19] , [36] , in this current case some amplitude modulation in Fourier space [37] is required for designing the loss-proof beam (see Supplementary Fig. 1 and discussion in the Supplementary Material for Fourier space analysis). The difference between generating the ordinary accelerating beam and launching the loss-proof beam is only at the tail, which in Fourier space is translated into diverging amplitude for the high positive wavevectors. We use a simple linear filter as a coarse amplitude mask, to impose the required Fourier space amplitude on the beam. The modulation profile for the linear filter is given by f ( x )=10 −(( N × OD )/(2 L )) x , where OD is the maximal optical density at the edge of the filter, L is the filter width and N is the number of filters used successively. In our experiment OD =4, L =45 mm and N =2, which is approximately equivalent to k ″= k ′/500. The beam is then demagnified and Fourier transformed using a × 60 microscope objective lens, to produce the accelerating beam in the spatial domain. We let the beam propagate in air and image its structure using a moving × 60 microscope objective and a CCD camera to capture its propagation dynamics. The results are shown in Fig. 4 , for acceleration parameter α =400. We compare between three types of beams: an ordinary non-paraxial accelerating beam ( Fig. 4a,b ), an exponentially growing accelerating beam ( Fig. 4c,d ), and an exponentially decaying accelerating beam ( Fig. 4e,f ). The latter, ‘gain-proof’ concept is very similar to loss-proof one but with opposite trends. Namely, the gain-proof beam is created with a wavevector containing a negative imaginary part: . This beam presents an ‘under-healing’ property rather than ‘over-healing’, and can propagate in gain media with no intensity amplification. In free space, the ‘gain-proof beam’ is shape-preserving while exhibiting exponential decay. Despite being less attractive for applications, the gain-proof beam is yet another demonstration of the counterintuitive results that accelerating beams provide—in this case, a shape-preserving beam which decays in free space and resists amplification. All three beams are created using an identical phase mask, and the only difference between them is their Fourier space amplitude, which is controlled through the amplitude mask. For the gain-proof beam, we flip the amplitude mask to apply the opposite profile: f ( x )=10 −(( N × OD )/(2 L ))( L − x ) . We find good agreement between the simulations and experiment, with a clear exponential growth (and decay) in intensity on the appropriate beams, while the ordinary accelerating beam is maintaining an approximately constant intensity value. The intensity grows by a factor of roughly 8 for the loss-proof beam, and decays by the same factor for the gain-proof beam. 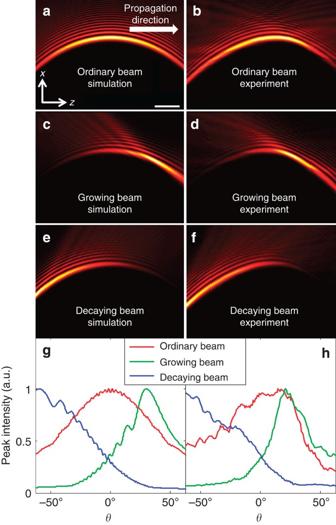Figure 4: Experiments comparing loss-proof, gain-proof and ordinary accelerating beams. (a) Simulated propagation dynamics of the ordinary non-paraxial accelerating beam (propagating from left to right). Scale bar, 10 μm. (b) Experimental results depicting the propagation dynamics of the ordinary accelerating beam. (c,d) Propagation dynamics of the exponentially growing beam, simulation and experiment. (e,f) Propagation dynamics of the exponentially decaying beam, simulation and experiment. (g) Simulated evolution of the peak intensity values for the ordinary accelerating beam (red), the exponentially growing beam (green) and the exponentially decaying beam (blue). (h) Experimental results showing the evolution of the peak intensity of the main lobe as a function of the bending angleθ. The ordinary accelerating beam maintains an approximately constant peak intensity for about 30 μm propagation, while the peak intensity of the loss-proof beam grows by a factor of 8, whereas the gain-proof beam decays by a factor of 8. Beam power is normalized. Figure 4: Experiments comparing loss-proof, gain-proof and ordinary accelerating beams. ( a ) Simulated propagation dynamics of the ordinary non-paraxial accelerating beam (propagating from left to right). Scale bar, 10 μm. ( b ) Experimental results depicting the propagation dynamics of the ordinary accelerating beam. ( c , d ) Propagation dynamics of the exponentially growing beam, simulation and experiment. ( e , f ) Propagation dynamics of the exponentially decaying beam, simulation and experiment. ( g ) Simulated evolution of the peak intensity values for the ordinary accelerating beam (red), the exponentially growing beam (green) and the exponentially decaying beam (blue). ( h ) Experimental results showing the evolution of the peak intensity of the main lobe as a function of the bending angle θ . The ordinary accelerating beam maintains an approximately constant peak intensity for about 30 μm propagation, while the peak intensity of the loss-proof beam grows by a factor of 8, whereas the gain-proof beam decays by a factor of 8. Beam power is normalized. Full size image To demonstrate some of the advantages of the loss-proof beam compared with an ordinary accelerating beam, we construct a setup designed to accelerate small polystyrene particles (diameter 10 μm) along a circular trajectory. The beam is shaped by a proper phase mask displayed on an SLM, and is accelerated through a cuvette filled with water which contains the 10 μm particles which are accelerated by the beam. In addition, the cuvette contains small diameter (50 nm) polystyrene particles which cause slight scattering and allow us to image the beam itself. The loss caused by scattering is negligible: α eff ≈0.02 mm −1 , so that the liquid is practically lossless. The light beam is accelerating the larger particles using the combination of the gradient force and radiation pressure. The water cuvette is imaged from above using a CCD camera, and allows us to track the particles as they scatter the incoming light. The particle tracks are recorded on video and analysed (see Supplementary Material for a video showing one experiment). 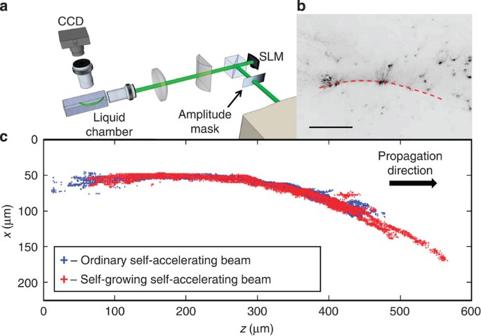Figure 5: Dynamics of microparticles accelerated on a circular trajectory by an accelerating beam. (a) Experimental setup. The predesigned Fourier space phase and amplitude are superimposed on a linearly polarized broad gaussian beam using an amplitude mask and a spatial light modulator (SLM). The beam size is adjusted using an imaging system composed of an f=250 mm cylindrical lens and an f=80 mm spherical lens. The beam is then Fourier transformed using a × 60 microscope objective, and launched to propagate through a liquid chamber. Polysterene microparticles (diameter 10 μm) are placed in the water-filled chamber driven by the incoming laser beam and imaged from above. (b) Typical image of the microparticles. The accelerating light beam is marked in red. Scale bar, 250 μm. (c) Comparison of the trajectories of the particles accelerated using the ordinary accelerating beam and the exponentially growing accelerating beam. Both beams have accelerating parameterα=1,600. Evidently, the particles accelerated using the growing beam ‘catch up’ with the light beam at a later phase, but then they stay on the bending beam and accelerate for longer distances and larger angles. The ordinary beam drives the particles up to 41° bending angle, while the loss-proof beam allows driving of particles up to 49°, which constitutes a 20% improvement in bending. Figure 5 shows a comparison of trajectories achieved using an ordinary accelerating beam and the loss-proof beam. Both beams carry the same total beam power of ~230 mW and the same phase profile with α =1,600; they only differ in their Fourier space amplitude. In this experiment, we use the same amplitude masking as in Fig. 4 , but with a single filter so as not to impair the total beam power. Figure 5 shows 14 trajectories of particles accelerated using the ordinary accelerated beam and 11 trajectories of particles accelerated using the loss-proof beam. The trajectories are superimposed one on top of the other. Both beams guide the microparticles to large non-paraxial angles, as opposed to the early pioneering experiments for which the design was strictly paraxial, hence the beams could accelerate the particles only to small angle bending (around 10 degrees), restricted by paraxiality [4] , [5] . The ordinary accelerating beam drives the particles on a circular trajectory up to 41° at most, after which the beam decays in power and cannot push the particles further. On the other hand, the loss-proof beam allows improved guiding, with trajectory bending as high as 49° before friction stops the particles. This presents an ~20% increase in trajectory length for the loss-proof beam, compared with the ordinary accelerating beam. Figure 5: Dynamics of microparticles accelerated on a circular trajectory by an accelerating beam. ( a ) Experimental setup. The predesigned Fourier space phase and amplitude are superimposed on a linearly polarized broad gaussian beam using an amplitude mask and a spatial light modulator (SLM). The beam size is adjusted using an imaging system composed of an f=250 mm cylindrical lens and an f=80 mm spherical lens. The beam is then Fourier transformed using a × 60 microscope objective, and launched to propagate through a liquid chamber. Polysterene microparticles (diameter 10 μm) are placed in the water-filled chamber driven by the incoming laser beam and imaged from above. ( b ) Typical image of the microparticles. The accelerating light beam is marked in red. Scale bar, 250 μm. ( c ) Comparison of the trajectories of the particles accelerated using the ordinary accelerating beam and the exponentially growing accelerating beam. Both beams have accelerating parameter α =1,600. Evidently, the particles accelerated using the growing beam ‘catch up’ with the light beam at a later phase, but then they stay on the bending beam and accelerate for longer distances and larger angles. The ordinary beam drives the particles up to 41° bending angle, while the loss-proof beam allows driving of particles up to 49°, which constitutes a 20% improvement in bending. Full size image In conclusion, we have presented the first loss-proof diffractionless accelerating beam. These are close-form shape-invariant accelerating solutions of Maxwell’s equations in the presence of linear and nonlinear absorption. We utilized these non-paraxial loss-proof accelerating beams experimentally, demonstrating applications in micromanipulation of particles in fluids, where these beams facilitate control over the particles over steeper angles than ordinary paraxial accelerating beams. The experiments presented here are also the first application of self-accelerating beams in non-paraxial micromanipulation of particles, displaying acceleration of microparticles at much steeper angles than ever achieved by optical means. The loss-proof and self-growing beams offer many interesting applications, such as long range loss-proof plasmons and abruptly focusing light beams in absorptive media. The latter is especially important in biological and medical applications such as multiphoton florescence microscopy, and improved control of optical manipulation of micro and nano-particles. The nonlinear loss-proof solutions presented here enable applications in highly nonlinear regimes, such as loss-proof light-induced curved plasma channels and a variety of other ideas related to nondiffracting beams propagating in lossy media, in principle—wherever light-matter interactions are dominant. The loss-proof concept is based solely on the self-healing property of nondiffracting beams, arising from interference effects. As such, it is a general concept that can be applied to other types of nondiffracting beams and other kinds of attenuation, including nonlinear losses, by defining the correct compensation rate from the tail of the beam. Furthermore, we expect that accurate design of the tail energy will allow controllable intensity profiles along propagation, including periodically growing and decaying light beams. We envision that the ability to arbitrarily predesign intensity patterns along the optical axis will pave the way to many new developments in the optical sciences. How to cite this article: Schley, R. et al. Loss-proof self-accelerating beams and their use in non-paraxial manipulation of particles’ trajectories. Nat. Commun. 5:5189 doi: 10.1038/ncomms6189 (2014).